Amplification of progenitors in the mammalian telencephalon includes a new radial glial cell type The mechanisms governing the expansion of neuron number in specific brain regions are still poorly understood. Enlarged neuron numbers in different species are often anticipated by increased numbers of progenitors dividing in the subventricular zone. Here we present live imaging analysis of radial glial cells and their progeny in the ventral telencephalon, the region with the largest subventricular zone in the murine brain during neurogenesis. We observe lineage amplification by a new type of progenitor, including bipolar radial glial cells dividing at subapical positions and generating further proliferating progeny. The frequency of this new type of progenitor is increased not only in larger clones of the mouse lateral ganglionic eminence but also in cerebral cortices of gyrated species, and upon inducing gyrification in the murine cerebral cortex. This implies key roles of this new type of radial glia in ontogeny and phylogeny. Ontogenetic mechanisms in the developing brain are the basis for the increase in neuron numbers in specific brain regions during phylogeny. For example, higher neuron numbers settling in the increased, often gyrated mammalian neocortex arise from increased progenitor numbers during development. These progenitors are accommodated in additional germinal layers, like the inner and outer subventricular zone (i/oSVZ) [1] , [2] , [3] , [4] that are located basal to the ventricular zone (VZ), where progenitors are anchored at the ventricular surface (VS). In most regions of the CNS, the vast majority of progenitor cells are within the VZ, where cells possess an epithelial polarity and comprise the stem cells of the developing nervous system, the neuroepithelial cells and later radial glia (RGs) [5] . These undergo interkinetic nuclear migration (INM), with the soma migrating during different phases of the cell cycle towards the apical VS, where M-phase takes place. It has therefore been suggested that the area of the VS may be limiting for the numbers of possible mitoses, and further increase of progenitor numbers is only possible by accommodating these at more basal positions, such as in the SVZ [2] , [6] . A further possibility that had been postulated is to allow cells maintaining the epithelial hallmarks of stem cells to undergo M-phase at non-apical positions, thereby overcoming the apical space limitations [2] . However, such a progenitor type has been elusive so far and the mechanisms of extended SVZ formation are still ill understood. Conversely, the cellular composition of the enlarged i/oSVZ has been unravelled in the recent years, and revealed a novel type of RG with long basal process, while lacking an apical anchoring, the basal radial glia (bRGs) [7] , [8] , [9] . These provide additional guiding structures for the higher neuronal numbers expanding the cerebral cortex surface in species with folded cerebral cortices (for reviews, see Borrell and Reillo [3] and Lui et al. [4] ). However, despite recent progress [10] , [11] , little is known about the cellular mechanisms involved in the generation of the bRGs and the expansion of the SVZ. In order to gain some insights into these processes, we examined the ventral telencephalon, the region of the murine brain with the largest SVZ. This region forms the ganglionic eminences (GE), two bulges (the lateral GE (LGE) and the medial GE (MGE)) protruding into the ventricle [6] . LGE progenitors generate striatal projection neurons and olfactory bulb interneurons [12] , [13] , that is, a particularly large number of neuronal progeny with the olfactory bulb interneurons continuing to be generated live long. Progenitors in the MGE also generate a large number of neurons, namely, most telencephalic interneurons migrating through the entire telencephalon except to the olfactory bulb, besides giving rise to projection neurons of the globus pallidus [14] , [15] . These regions are thus well suited to examine the mechanisms of enlarging the number of SVZ progenitors and subsequent neuronal progeny. By live imaging of brain slices and immunostaining of mitotic cells in the GE, we here discover a novel progenitor type dividing within the VZ but at subapical positions. This includes cells with RG morphology, that is, a bipolar (bp) morphology with a basal and apical process visible during the M-phase, as previously predicted [2] . Such bpRGs are also present in the VZ but are further extended into the i/oSVZ of species with gyrated cerebral cortices. Consistent with their role in amplifying neuron numbers, they are enriched in larger clones generated in the murine ventral telencephalon and the cerebral cortex when gyrification is elicited. A majority of non-apical progenitors in the developing GE While most progenitor cells divide at the apical surface (apical progenitors, AP) during brain development, this is strikingly different in the GE, where basally dividing cells (PH3+) gradually outnumber APs, reaching 60–70% in the LGE and MGE, respectively ( Fig. 1a ). We also noted non-surface mitoses within the VZ [6] (Fig. 1c) , the zone of AP INM covering a distance of 11 cell diameters determined by live imaging ( Supplementary Fig. S1a ). These subapical progenitors (SAPs) ( Fig. 1c ) increase from 7% (LGE) and 10% (MGE) at E14 to over 20% of all mitoses at E16 in both these regions ( Fig. 1d ). Among the mitoses within the VZ, SAPs reached 47% in LGE and 54% in the MGE at E16. Conversely, mitoses at subapical or basal positions remained a minority throughout neurogenesis in the dorsal telencephalon ( Fig. 1b ). 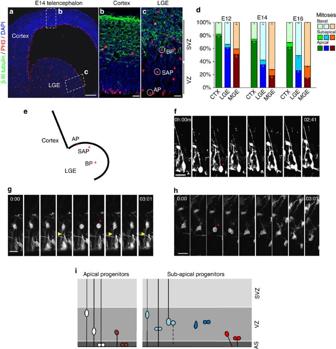Figure 1: Distribution of mitotic cells in the ventral telencephalon shows a dominance of non-apical mitoses. (a–c) Fluorescence micrographs of E14 mouse telencephalon sections immunostained for phosphorylated histone H3 (PH3, cells in mitosis) and βIII-tubulin (neurons) show the predominance of progenitors dividing apically (AP) in the dorsal telencephalon (cortex ina,b) in contrast to an abundance of non-apical mitoses comprising BP in the SVZ and cells dividing at subapical positions (SAP) within the VZ (c) in the lateral ganglionic eminence (LGE ina,c). (d) Histograms depicting the proportion of PH3+ cells dividing at the respective positions (cerebral cortexn=1,201 cells (E12), 1,498 (E14), 879 (E16); LGE: 594 (E12), 1,569 (E14), 1,069 (E16), three animals at each timepoint; data are mean±s.e.m.; MGE: 1145 (E12), 1632 (E14), 1632 (E16)). (e) Scheme depicting the position of cells observed in mitosis at different positions (fapical,gsubapical,hbasal, red asterisks) by live imaging, with yellow arrowheads depicting processes (apical ing). Time is depicted in hours (h) and minutes (m). (i) Scheme illustrating the different VZ progenitor types (APs and SAPs) present in the LGE. Scale bars, 100 μm (a), 10 μm (b), 20 μm (f–h). Figure 1: Distribution of mitotic cells in the ventral telencephalon shows a dominance of non-apical mitoses. ( a – c ) Fluorescence micrographs of E14 mouse telencephalon sections immunostained for phosphorylated histone H3 (PH3, cells in mitosis) and βIII-tubulin (neurons) show the predominance of progenitors dividing apically (AP) in the dorsal telencephalon (cortex in a , b ) in contrast to an abundance of non-apical mitoses comprising BP in the SVZ and cells dividing at subapical positions (SAP) within the VZ ( c ) in the lateral ganglionic eminence (LGE in a , c ). ( d ) Histograms depicting the proportion of PH3+ cells dividing at the respective positions (cerebral cortex n =1,201 cells (E12), 1,498 (E14), 879 (E16); LGE: 594 (E12), 1,569 (E14), 1,069 (E16), three animals at each timepoint; data are mean±s.e.m. ; MGE: 1145 (E12), 1632 (E14), 1632 (E16)). ( e ) Scheme depicting the position of cells observed in mitosis at different positions ( f apical, g subapical, h basal, red asterisks) by live imaging, with yellow arrowheads depicting processes (apical in g ). Time is depicted in hours (h) and minutes (m). ( i ) Scheme illustrating the different VZ progenitor types (APs and SAPs) present in the LGE. Scale bars, 100 μm ( a ), 10 μm ( b ), 20 μm ( f – h ). Full size image Live imaging of progenitor cells in slices of the LGE To unravel how these progenitor types dividing at different positions are lineally related, we performed live imaging of cells labelled with GFP-expressing plasmids by in utero electroporation (IUE) at E13. In slices of the LGE prepared 24 h later, we observed two types of APs ( Fig. 1e ) that undergo INM and mitosis at the VS: the classical RGs with a bipolar morphology encompassing a long radial process and an apical process reaching the VS that divide at the apical surface, with only their basal process visible in M-phase ( Fig. 1f ), and the ‘short neural precursor cells’ (SNPs) [16] , [17] , [18] that lack a longer basal process but possess an apical process, also undergoing INM and dividing at the VS without any process visible in M-phase ( Fig. 2a , Supplementary Fig. S1b ). Some cells with only an apical process did not reach the apical surface for mitoses but divided at some distance from the ventricle, at subapical positions ( Fig. 1g , yellow arrowhead highlighting the apical process; Supplementary Movie 1 ). We also detected RGs with both apical and long basal processes during M-phase, dividing at subapical positions ( Supplementary Fig. S1c ; white arrowhead in scan through z-stack in Supplementary Movie 2 ). Some cells dividing at subapical positions within the VZ had only short processes and retracted these processes in M-phase, being entirely round and thus morphologically resembling basal progenitors (BPs) ( Figs 1h and 2 ). While cells dividing within the VZ at apical or subapical positions were heterogeneous in their morphology, most cells dividing at further basal positions were multipolar in morphology, lacking any longer apical or basal contact resembling classical BPs ( Fig. 1h ) as described originally in the neocortex [5] . Thus, the novel population of SAPs is heterogeneous, comprising cells with only an apical process, both apical and basal processes or no longer processing in M-phase (summarized in Fig. 1i ). 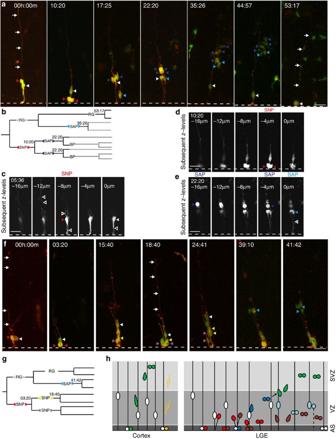Figure 2: Live imaging of apical progenitors and their progeny in the LGE. (a) Time-lapse series of a clone consisting of a RG (white arrowhead) and a SNP (lacking a basal process, red arrowhead). The SNP divides at the ventricle (dashed white line; two red arrowheads indicate M-phase) (t:10:20), giving rise to two SAPs (dark blue arrowheads) that divide again in the VZ (t:22:20). The RG also divides at the ventricle, giving rise to a RG and a SAP (white and blue arrowhead in t:17:25) that divides in the VZ (two blue arrowheads in t:35:26), whereas the RG undergoes mitosis at the ventricle (t:53:17; white arrowheads: basal process of RG). (b) Lineage diagram derived from the time-lapse movie in (a); note that BPs continued to proliferate in the SVZ, but could not be individually followed due to their fast movement and decreased GFP signal (dashed lines). Note that the length of the lines in (b) and (g) are not drawn to scale (time). (c–e) Single optical sections from z-stacks reveal details of the respective imaging timepoints indicated. Full arrowheads point to the cell body of progenitor cells and white outlined arrowheads point to the respective processes of cells. For example, the short basal and apical process of the SNP in (a) are shown in (c) at a different timepoint. (f) Time-lapse series illustrating the generation of multiple VZ progenitors coming from a single labelled cell. The SNP divides at the ventricle (red arrowheads; t:03:20), giving rise to two SNPs that divide again at the ventricle (red arrowheads at t:18:40). The RG (white arrowhead in t:03:20) gives rise to one RG and one SAP that divides between t:39:10 and t: 41:42 (blue arrowheads). (g) Lineage diagram derived from the time-lapse series in (f). Note that the two daughter SNPs generated by a SNP (red) divide at a very similar time point at the ventricle. Scale bars, 20 μm (a,d,c,e,f). (h) Scheme illustrating the progenitor lineage detected in the LGE in comparison with the neocortex. For a print-out of this figure please refer toSupplementary Fig. 9with adjusted gamma value and both channels combined in grayscale to maintain the visibility of fine processes. Figure 2: Live imaging of apical progenitors and their progeny in the LGE. ( a ) Time-lapse series of a clone consisting of a RG (white arrowhead) and a SNP (lacking a basal process, red arrowhead). The SNP divides at the ventricle (dashed white line; two red arrowheads indicate M-phase) (t:10:20), giving rise to two SAPs (dark blue arrowheads) that divide again in the VZ (t:22:20). The RG also divides at the ventricle, giving rise to a RG and a SAP (white and blue arrowhead in t:17:25) that divides in the VZ (two blue arrowheads in t:35:26), whereas the RG undergoes mitosis at the ventricle (t:53:17; white arrowheads: basal process of RG). ( b ) Lineage diagram derived from the time-lapse movie in ( a ); note that BPs continued to proliferate in the SVZ, but could not be individually followed due to their fast movement and decreased GFP signal (dashed lines). Note that the length of the lines in ( b ) and ( g ) are not drawn to scale (time). ( c – e ) Single optical sections from z-stacks reveal details of the respective imaging timepoints indicated. Full arrowheads point to the cell body of progenitor cells and white outlined arrowheads point to the respective processes of cells. For example, the short basal and apical process of the SNP in ( a ) are shown in ( c ) at a different timepoint. ( f ) Time-lapse series illustrating the generation of multiple VZ progenitors coming from a single labelled cell. The SNP divides at the ventricle (red arrowheads; t:03:20), giving rise to two SNPs that divide again at the ventricle (red arrowheads at t:18:40). The RG (white arrowhead in t:03:20) gives rise to one RG and one SAP that divides between t:39:10 and t: 41:42 (blue arrowheads). ( g ) Lineage diagram derived from the time-lapse series in ( f ). Note that the two daughter SNPs generated by a SNP (red) divide at a very similar time point at the ventricle. Scale bars, 20 μm ( a , d , c , e , f ). ( h ) Scheme illustrating the progenitor lineage detected in the LGE in comparison with the neocortex. For a print-out of this figure please refer to Supplementary Fig. 9 with adjusted gamma value and both channels combined in grayscale to maintain the visibility of fine processes. Full size image Given this heterogeneity in progenitor subtypes, we were interested to determine how these progenitor types are connected to each other during lineage progression. We approached this by using sparse clonal labelling [10] by plasmids containing Cre and 2 reporters behind a floxed stop cassette containing cytoplasmic GFP and a membrane-tagged Kasabian orange to visualize all cellular processes (see Supplementary Fig. S1d,e for examples of AP and BP morphology in M-phase). To ensure full process visualization, we imaged in the centre of the slice and started with a RG cell with its long fully-intact basal processes not reaching any of the cut surfaces ( Supplementary Movie 3 ). This revealed a profoundly larger progeny of RGs within 48–56 h compared with the pattern of cell divisions reported for the neocortex at similar developmental stages [19] , as almost all daughter cells of RGs continued to divide and no postmitotic cells emerged directly from the apically dividing RGs in the LGE ( Fig. 2 and Supplementary Fig. S2a ). Moreover, this extended imaging time revealed a consistent sequence among the diverse progenitor types progressing from APs over SAPs to BPs ( Fig. 2 ). An apically dividing RG always self-renewed and generated besides itself either an apically dividing SNP or a SAP ( Fig. 2a and Supplementary Fig. S2a ). These SNPs could either generate further SNPs or SAPs and the SAPs could in turn generate SAPs or basally dividing BPs, thereby mediating the lineage progression from apical (RGs and SNPs) through subapical to basal positions ( Fig. 2a–h and Supplementary Fig. S2a ). Notably, virtually all clones retained an apically dividing radial glia ( Fig. 2a ), the self-renewing ancestor of the amplifying intermediates. A series of proliferative amplifying progenitors in the LGE Importantly, this lineage observed by live imaging revealed various cellular mechanisms of amplifying progenitor numbers. This included several proliferative, amplifying steps still within the VZ. In most cases, the direct progeny of apically dividing RGs divided again in the VZ (45/52 cells; Fig. 2 ; Supplementary Movies 4 and 5 ). These were either APs consisting of RGs or SNPs (SNP; red arrowhead in Fig. 2a t:10:20) or SAPs ( Fig. 2a t: 35:26). Notably, SNPs also generated daughter cells that further proliferated within the VZ either as SNPs dividing at the apical surface ( Fig. 2f ) or as SAPs dividing at subapical positions ( Fig. 2a ). This is rather different from the cerebral cortex, where SNPs in majority directly generate postmitotic neurons [16] , [17] , [18] and SAPs had not been observed before. Progenitor amplification continued further with SAPs that generated, in most cases (64%, Supplementary Fig. S2b ), daughter cells undergoing further divisions ( Fig. 2a and Supplementary Movie 4 ). This continuous generation of proliferative daughters in the LGE, first in the VZ at apical and subapical positions, and then in the SVZ, could result in as many as 11 daughter cells within 48 h of observation ( Supplementary Movie 6 and Fig. 2a ; 10 cells within 53 h). Additionally, we also detected proliferative divisions of BPs in the SVZ ( Supplementary Fig. S3a and Supplementary Movie 7 ), rather than undergoing terminal divisions as in the cerebral cortex [19] , [20] , [21] . Thus, live imaging of progenitors in the LGE revealed several rounds of proliferative divisions at various positions, including a novel type of progenitor dividing at subapical locations within the VZ. Cell cycle shortening in subsequent progenitor divisions Live imaging further revealed a continuously faster cell cycle with each progenitor generation ( Supplementary Fig. S2c ). RGs had the longest cell cycle length (25 h mean), whereas their first daughter cells, the apically dividing SNPs or the SAPs, had a mean cell cycle length of 17 h ( Supplementary Fig. S2c,d ). The second-generation SAPs emerging from either SNPs or SAPs had a significantly shorter cell cycle of about 12 h ( Supplementary Fig. S2d ). Thus, independent of the progenitor subtype, the cell cycle length shortened with each generation in the LGE ( Supplementary Fig. S2c ), whereas it increased in cortical BPs imaged under the same conditions ( Supplementary Fig. S2e ; see also Arai et al. [22] ). Taken together, besides a series of proliferative divisions the continuously faster cell cycle of the progeny serves to amplify the number of progeny generated in a given time—both hallmarks of the adult neural stem cell lineages [23] emerging from this region. SAPs are enriched in larger LGE clones However, not all cells observed by live imaging of the LGE generated a large number of progeny (see Supplementary Movie 8 ). In a total of 52 lineages observed live, the number of daughter cells ranged from 2 to 11 ( Fig. 3a ), with clones of either size distributed randomly along the dorsal to ventral axis of the LGE ( Fig. 3b ), thus lacking a preferential location suggestive of a particular neuronal progeny [13] . While the SAP-containing lineages also showed no specific spatial location, we noted a striking bias of SAPs contributing virtually always to larger clones (clone size ≥5, 90%, n =21), whereas smaller size lineages (clone size <5) contained SAPs only in a minority of cases (29%, n =31). Thus, the presence of SAPs clearly predicts amplification of the progeny typically occurring in the lineage branch comprising the SAPs ( Supplementary Fig. S2a ). These data suggest that this novel progenitor type serves to amplify the progeny of RGs in the LGE, starting already in the VZ. 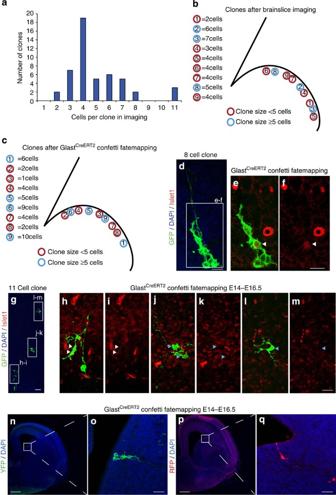Figure 3: Progenitors of different proliferative behaviour contribute to the striatal projection neuron lineage in the LGE. (a) Summary of clone sizes observed by live imaging (48–62 h) distributed as exemplified in the drawing in (b) for one imaging experiment (three slices). (c) Distribution of clones observed by genetic fate mappingin situwith micrographs of two examples of clones doublestained for Islet1 (red) (white arrowheads: double-positive cells; blue arrowheads: Islet1-negative cells) depicted in (d–m). (n–q) Examples of clonally labelled cells induced by TM in GlastCreERT2Confetti reporter mice at E14. Scale bars, 200 μm (f,g), 50 μm (e), 20 μm (d,f,m,n–q). Figure 3: Progenitors of different proliferative behaviour contribute to the striatal projection neuron lineage in the LGE. ( a ) Summary of clone sizes observed by live imaging (48–62 h) distributed as exemplified in the drawing in ( b ) for one imaging experiment (three slices). ( c ) Distribution of clones observed by genetic fate mapping in situ with micrographs of two examples of clones doublestained for Islet1 (red) (white arrowheads: double-positive cells; blue arrowheads: Islet1-negative cells) depicted in ( d – m ). ( n – q ) Examples of clonally labelled cells induced by TM in Glast CreERT2 Confetti reporter mice at E14. Scale bars, 200 μm ( f , g ), 50 μm ( e ), 20 μm ( d , f , m , n – q ). Full size image Characterization of SAPs in the LGE in situ In order to determine the morphological heterogeneity of SAPs observed by live imaging in slices, also in situ, we first examined to what extent immunostaining for the phosphorylated form of vimentin (p-vimentin) reliably labels the major processes of mitotic cells [24] . Immunostaining 31 h after electroporation with a plasmid encoding a membrane-anchored form of GFP (plox-eGFP-farnesylated) showed that p-vimentin labelled in almost all cases the major processes of cells in mitoses (for examples of APs, SAPs and BPs see Supplementary Fig. S4a-c ; for 3D reconstructions see Supplementary Movie 9 ). P-vimentin+ cells at subapical positions were relatively frequent in the GE and exhibited a single major process directed either apically ( Supplementary Fig. S4d , green arrow, 13%) or basally ( Supplementary Fig. S4e , 7%), or were bipolar in M-phase with a major apical and basal process reminiscent of the subapically dividing RGs ( Supplementary Fig. S4f, 24 %; 3D reconstruction in Supplementary Movie 10 ). In addition, we also observed 55% of p-vimentin+ cells at subapical positions lacking any major process labelling in M-phase ( Supplementary Fig. S4d , yellow arrow). Thus, p-vimentin staining revealed a similar morphological heterogeneity of mitotic cells at subapical positions as that observed by live imaging, including a population with RG morphology. Accordingly, some SAPs were also immunopositive for radial glia markers, such as RC2 ( Supplementary Fig. S4g ), GLAST ( Supplementary Fig. S4h ) and hGFAP-GFP [25] ( Supplementary Fig. S4i ). Interestingly, SAPs were rarely positive for BLBP, which was confined to apically dividing radial glia ( Supplementary Fig. S4j ), but expressed Sox2, Dlx2, Pax6 and Ascl1 ( Supplementary Figs S4k , S5a,b and S8a–c ), well-known transcription factors in LGE progenitors. Clonal heterogeneity in the LGE in situ Next we aimed to examine the clone size in situ for comparison with the lineage size observed within 40–56 h by live imaging in slices. Towards this aim, we induced genetic recombination in a single RG in vivo by low doses of tamoxifen (5 μg g −1 ) in GLAST CreERT2 mice crossed to the multicolour reporter line Confetti [26] . Analysis of the progeny was performed at a comparable time interval of 2–3 days later. As no cluster contained cells of different colours ( n =62), the distinct clusters of cells labelled by the same fluorescent protein are considered as clones ( Fig. 3c–q ). Comparable to the live imaging data, clones comprised 2–10 cells ( n =62) and clones of different sizes were distributed broadly within the LGE ( Fig. 3c ) as observed by imaging in slices ( Fig. 3b ). The transcription factor Islet1 begins to be expressed in differentiating striatal projection neurons [13] . Islet1-immunoreactive cells were already observed in about 25% of all clones (10 of 42 clones) 63 h after induction of recombination in RGs. Most of these (80%) comprised more than 5 cells including larger clones with 11, 8 and 15 cells ( Fig. 3d–m ). Likewise, staining of slices post imaging revealed a daughter cell of a subapically dividing RG beginning to acquire Islet1 ( Supplementary Fig. S5c ,d). Thus, the heterogeneity of clones, including a contribution to the striatal lineage and the generation of up to 10 daughter cells within 48–56 h, was confirmed in situ . SAPs in the VZ and SVZ of gyrated cortices As the above analysis implied SAPs in the amplification of daughter cells in several brain regions and lineages, such as striatal neurons in the LGE and the lineage derivatives from the MGE ( Fig. 1d ), we next asked to what extent SAPs may also be relevant for the expansion of other brain regions, such as gyrated cerebral cortices in other mammalian species [4] , [27] . Indeed, PH3+ cells at subapical positions were present in the VZ of the ferret cerebral cortex at postnatal day 2 (P2), accounting for 30% of all VZ divisions by P6 ( Fig. 4a ). Virus-GFP labelling revealed a morphological heterogeneity of cells in the VZ and iSVZ, with some having both basal and apical processes likely resembling the subapically dividing RGs in the murine LGE VZ ( Fig. 4d ). P-vimentin staining of mitotic cells confirmed this heterogeneity, with bipolar cells bearing apical and basal processes in M-phase and others having only one process, either apical or basal ( Fig. 4c ). Strikingly, RG-like p-vimentin+ cells with a basal and apical process extended also into the iSVZ and, to some extent, even to the oSVZ ( Fig. 4c ), that is, far beyond the regions where these cells were observed in the mouse (see also virus-GFP-labelled bipolar cells in Fig. 4f ). Thus, bipolar RGs (bpRGs) dividing at non-apical positions can be detected not only in the VZ, but also in the iSVZ/oSVZ of the ferret. As these do not divide at subapical positions within the VZ, we refer to these more globally as bpRGs, thereby discriminating them from bRGs with only a basally oriented process ( Fig. 4h ) and apical RGs dividing at the VS. 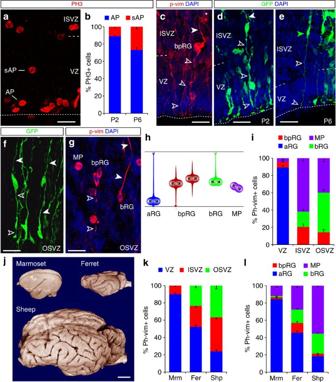Figure 4: Distribution of mitotic cells in the neocortex of gyrencephalic species shows a high abundance of bipolar radial glia. (a,c–g) Fluorescence micrographs of ferret neocortex sections (postnatal day 2, P2 (c,d,f,g) and P6 (e) immunostained as indicated (phosphorylated histone H3=PH3; phosphorylated-vimentin=p-vim)), showing mitotic apical (AP) and subapical progenitors (SAP) within the VZ and ISVZ (a,c–e) and OSVZ (f,g). Progenitor cells in ISVZ and OSVZ displaying the typical morphology of bpRGs with a basal process (solid arrowheads) and a long apical process (open arrowheads) were revealed by Rv:gfp(d,f) or Adeno-gfpinjection (e) or p-vim (c,g). Note also bRGs with only a basal process and multipolar progenitors (MP) without longer processes. Schematic drawings in (h) depict the defining characteristics of the different progenitor cell types analysed in the species indicated in (j); external view of the adult brains at scale. Histograms in (b,i,k,l) depict AP and bpRG, MP and bRG mitoses in the ferret VZ at P2 and P6 (b),n=982, 250, respectively (three animals each), proportions of the cell types indicated in (h) defined by p-vim in P2 ferret neocortex (i),n=623 cells in VZ, 290 ISVZ, 277 OSVZ (three animals), and in all germinative layers (l), the contribution of which is shown in (k), in the marmoset (Mrm), ferret (Fer) and sheep (Shp) at equivalent stages of cortical development (E85, P2, E65–67, respectively; marmoset,n=1,743 cells; ferret, 1,190 cells; sheep, 2,435 cells; three subjects of each species). Data are mean±s.e.m. Scale bars, 20 μm (a,c,d,f,g); 40 cm (e); 1 cm (j). Figure 4: Distribution of mitotic cells in the neocortex of gyrencephalic species shows a high abundance of bipolar radial glia. ( a , c – g ) Fluorescence micrographs of ferret neocortex sections (postnatal day 2, P2 ( c , d , f , g ) and P6 ( e ) immunostained as indicated (phosphorylated histone H3=PH3; phosphorylated-vimentin=p-vim)), showing mitotic apical (AP) and subapical progenitors (SAP) within the VZ and ISVZ ( a , c – e ) and OSVZ ( f , g ). Progenitor cells in ISVZ and OSVZ displaying the typical morphology of bpRGs with a basal process (solid arrowheads) and a long apical process (open arrowheads) were revealed by Rv: gfp ( d , f ) or Adeno- gfp injection ( e ) or p-vim ( c , g ). Note also bRGs with only a basal process and multipolar progenitors (MP) without longer processes. Schematic drawings in ( h ) depict the defining characteristics of the different progenitor cell types analysed in the species indicated in ( j ); external view of the adult brains at scale. Histograms in ( b , i , k , l ) depict AP and bpRG, MP and bRG mitoses in the ferret VZ at P2 and P6 ( b ), n =982, 250, respectively (three animals each), proportions of the cell types indicated in ( h ) defined by p-vim in P2 ferret neocortex ( i ), n =623 cells in VZ, 290 ISVZ, 277 OSVZ (three animals), and in all germinative layers ( l ), the contribution of which is shown in ( k ), in the marmoset (Mrm), ferret (Fer) and sheep (Shp) at equivalent stages of cortical development (E85, P2, E65–67, respectively; marmoset, n =1,743 cells; ferret, 1,190 cells; sheep, 2,435 cells; three subjects of each species). Data are mean±s.e.m. Scale bars, 20 μm ( a , c , d , f , g ); 40 cm ( e ); 1 cm ( j ). Full size image To test for a correlation in the frequency of bpRGs and the gyrification index (GI) of the cerebral cortex, we examined the cerebral cortex of a near-lissencephalic primate, the marmoset [28] , [29] , and a mammal with a particularly high GI, the sheep [9] , [30] ( Fig. 4j ), at equivalent stages of cortical development [9] , [28] . Within the VZ, SAPs were very infrequent in both marmoset (2%) and sheep (1%). However, only about 10% of all mitotic p-vimentin+ cells were located in the SVZ of the marmoset, whereas nearly 80% were located there in the sheep embryo ( Fig. 4k ). Thus, the number of bpRGs was quite large in the developing sheep neocortex even though their proportion is outnumbered by bRGs and BPs ( Fig. 4l ). Importantly, both bpRGs and bRGs were less than 4% of all cortical progenitors in the marmoset, whereas they comprise nearly 30% of the progenitor pool in the sheep at equivalent stages ( Fig. 4l and Supplementary Fig. S6a ). Thus, RGs with a bipolar morphology in M-phase dividing at subapical or further basal positions are more abundantly present in the developing cerebral cortex of species with higher gyrification. Subapically dividing RGs generate bRGs in mouse LGE Given the above observations, we next examined whether bpRGs dividing non-apically may generate bRGs that have been shown to be a key cell type in gyrification (for reviews, see Borrell and Reillo [3] and Lui et al. [4] ). Indeed, we readily observed subapical RGs dividing asymmetrically, with a basal daughter cell maintaining the long basal process and an apical daughter cell inheriting the apical process ( Supplementary Fig. S7a,b ; Supplementary Movie 11 ; for scan through the z-stack of the mitotic subapical RGs in Supplementary Fig. S7b , see Supplementary Movie 3 ). These bRG daughter cells then moved further basally and divided within the SVZ ( Supplementary Fig. S7a ,b), sometimes twice ( Supplementary Fig. S7c ). Notably, both basal and subapically dividing RGs showed the characteristic pattern of initially apically-directed movements, followed by a fast basal movement and subsequent mitosis ( Supplementary Fig. S7b , see also Hansen et al. [7] , Shitamukai et al. [10] and Wang et al. [31] ). Thus, besides acting as a further amplification step in the progeny amplification in the LGE, SAPs, in particular the subapically dividing RGs, generate bRGs, a key cell type for expansion and folding of the mammalian cerebral cortex. Subapically dividing RGs increase upon Trnp1 knockdown This then allowed us to investigate the emergence of subapically dividing RGs in a recent model of gyrification in the murine cerebral cortex [11] . Knockdown of Trnp1 in the mouse cerebral cortex not only results in radial expansion and often folding of the electroporated region [11] , but also an expanded SVZ after 24 h ( Fig. 5a ). Given the expansion of the SVZ including 3x increased bRGs in this experimental model, we used live imaging to assess the abundance of bipolar subapically dividing RGs, the cell type directly generating bRGs in the GE. GFP+ cells were examined 24 h after electroporation with either a control vector or the shTrnp1 vector by immunohistochemistry for their bipolar morphology with longer basal and apical GFP+ processes during mitosis (PH3+) at non-apical positions ( Fig. 5b ). As expected, virtually no such cells could be detected with the control plasmid, whereas 20% of such cells were detected after knockdown of Trnp1 ( Fig. 5c ). Excitingly, these subapically dividing RGs could readily be observed in live imaging experiments starting 48 h after IUE in slices prepared 24 h after Trnp1 knockdown in the cerebral cortex ( Fig. 5d ). Interestingly, they recapitulated the behaviour described above for their counterparts in the LGE, with an initial apically directed movement (first hour in Fig. 5d ), but undergoing cell division at subapical positions, that is, prior to reaching the apical surface, generating a basally translocating daughter bRG. Thus, Trnp1 knockdown further links the frequency of subapically dividing RGs to the emergence of bRGs and the extended SVZ even in the murine cerebral cortex. 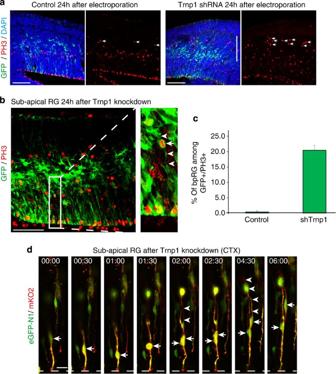Figure 5: The number of bipolar subapically dividing RGs is increased in Trnp1-shRNA electroporated cells in the developing mouse cerebral cortex. (a) Fluorescent micrograph of a section of embryonic day 14 cerebral cortex 24 h afterin uteroelectroporation with either control plasmid (left) or Trnp1-shRNA-GFP plasmid (right). Note the expanded DAPI-dense OSVZ-like region (indicated by the white line in the third panel) with many proliferating (PH3+) cells (indicated by white arrows). (b) Subapical RGs after Trnp1 knockdown identified by PH3 (red) and bipolar morphology in M-phase (white arrows pointing to green, GFP-labelled processes). (c) Quantification of bipolar-GFP+/PH3+ RGs dividing at non-apical positions among all GFP+/PH3+ cells after Trnp1 knockdown in comparison with the control (controln=159 cells; Trnp1-shRNAn=203 cells, three animals in each condition; error bars are s.e.m.). (d) Still frames of a movie of a subapically dividing RG imaged 48 h after Trnp1-shRNA electroporation. Note the characteristic apically directed movement before dividing at subapical position (arrows point to cell somata, arrowheads towards the long basal process). Scale bars 100 μm (a,b), 20 μm (d). Figure 5: The number of bipolar subapically dividing RGs is increased in Trnp1-shRNA electroporated cells in the developing mouse cerebral cortex. ( a ) Fluorescent micrograph of a section of embryonic day 14 cerebral cortex 24 h after in utero electroporation with either control plasmid (left) or Trnp1-shRNA-GFP plasmid (right). Note the expanded DAPI-dense OSVZ-like region (indicated by the white line in the third panel) with many proliferating (PH3+) cells (indicated by white arrows). ( b ) Subapical RGs after Trnp1 knockdown identified by PH3 (red) and bipolar morphology in M-phase (white arrows pointing to green, GFP-labelled processes). ( c ) Quantification of bipolar-GFP+/PH3+ RGs dividing at non-apical positions among all GFP+/PH3+ cells after Trnp1 knockdown in comparison with the control (control n =159 cells; Trnp1-shRNA n =203 cells, three animals in each condition; error bars are s.e.m.). ( d ) Still frames of a movie of a subapically dividing RG imaged 48 h after Trnp1-shRNA electroporation. Note the characteristic apically directed movement before dividing at subapical position (arrows point to cell somata, arrowheads towards the long basal process). Scale bars 100 μm ( a , b ), 20 μm ( d ). Full size image Ascl1 expression and role in SAPs To determine the molecular mechanisms regulating the higher numbers of SAPs in the murine LGE, we examined the transcription factor Ascl1, as it regulates progenitor amplification in this region [32] . As all SAPs were Ascl1+ ( Supplementary Fig. S8a–c ), its functional role was determined by Cre and control plasmid electroporation into the LGE of Ascl1 fl/+ and fl/fl embryos at E12. Interestingly, the proportion of GFP+ APs (PH3+ at the ventricular surface) examined 2 days later was not affected by the loss of Ascl1, whereas SAPs and BPs were significantly reduced in number ( Supplementary Fig. S8e,f ). Notably, Ascl1 immunoreactivity was also observed in about 30% of bipolar p-vimentin+ cells in the VZ, iSVZ and oSVZ of the ferret cerebral cortex ( Supplementary Fig. S6b,c ), consistent with Ascl1+ cells in VZ, iSVZ and oSVZ of the developing human cerebral cortex [33] , implying Ascl1 in the amplification of non-apical progenitors in various species and brain regions. Taken together, in this study we unravelled several cellular mechanisms contributing to SVZ enlargement in the murine ventral telencephalon and discovered a novel population of progenitors amplifying the progenitor pool in a radial dimension. This involves progenitors that still divide within the VZ but do not return to the apical surface for mitosis, and rather divide at subapical positions. Some of these maintain an apical process and some even possess full RG morphology with both apical and basal processes and undergo mitosis at subapical positions. Intriguingly, such a progenitor cell had been predicted [2] to allow progenitor expansion beyond a limited apical surface [6] , and is indeed particularly frequent in developing gyrated cerebral cortices as in ferret and sheep. Interestingly, in these species, RGs with a bipolar morphology in M-phase even extend beyond the VZ into i/oSVZ and thus further amplify in numbers. In summary, we provide four different lines of evidence linking the novel progenitor subset to SVZ and neuronal lineage amplification: (a) they are highly enriched in lineages of the murine LGE generating more than five daughter cells within 40–50 h of observation; (b) they are reduced in number in the murine LGE when SVZ expansion is decreased by deletion of Ascl1; (c) they are potently increased in number in the murine cerebral cortex when the SVZ is expanded by knockdown of Trnp1 and (d) they are increased in number in developing gyrated cerebral cortices of ferrets and sheep. Thus, SAPs are present in various forebrain regions, but their numbers significantly increase when radial expansion occurs and the number of neurons generated per time is increased. Moreover, we showed subapically dividing RGs to generate basal RGs, a cell type thought to be crucial for the expansion of the cerebral cortex in gyrification [3] , [4] , suggesting that the former contribute to expand bRGs beyond the limitations of the ventricular surface, eventually leading to the hugely expanded i/oSVZ in animals with gyrified cortices [2] , [4] , [9] . Apically anchored, but subapically dividing cells may thus represent the first steps in overcoming the limitation of the apical surface, allowing further expansion of RG lineages in a non-linear fashion and thereby enabling (radial) expansion of specific brain regions. Continuous live imaging of LGE progenitor cells further revealed general principles of generating an enlarged SVZ and neuronal output. In contrast to the cerebral cortex, shortening of cell cycle length occurs in subsequent intermediate progenitor cell divisions in the LGE (SNPs, SAPs, BPs), generating a larger number of progeny within a given time period. This differs from most observations in embryonic neurogenesis with subsequent rounds of division typically decreasing cell cycle speed. A second principle of lineage amplification emerging from live imaging in the LGE is repetitive proliferative divisions of all progenitor types. Importantly, both of these amplifying mechanisms are reminiscent of transient amplifying progenitors observed with a faster cell cycle in the adult neural stem cell lineages [23] , and may predispose this region to contribute to such a lineage in the adult brain. In this regard, the clear hierarchy among the different progenitor cell types is also important. Radial glia always divided asymmetrically, with distinct daughter cell fates generating one branch amplifying the lineage and the other branch self-renewing themselves (see examples in Supplementary Fig. S2a ). Thus, in the mouse LGE, the only self-renewing stem cells are apically dividing RGs, the founder cells of a clear hierarchy of further amplifying progenitors. The first progenitors generated from apical RGs are often SNPs, which we could observe to originate from RGs. Moreover, SNPs give rise to further amplifying progenitors in the LGE, rather than generating postmitotic neurons as suggested for murine cortical SNPs [17] , [18] , thereby also contributing to lineage amplification. However, their presence is not restricted to the larger clones (≥5 cells), but SNPs also occur frequently in smaller lineages observed in the LGE (see Supplementary Fig. S2a ). Importantly, this is not the case for SAPs that were largely confined to lineages with larger progeny (≥5 cells). SAPs arise either from SNPs as a second intermediate progenitor type, or directly from apical RGs. SAPs proliferate further and generate an enlarged number of BPs and bRGs, the cell types forming the SVZ. BPs in the LGE often undergo proliferative divisions, thereby expanding the pool of SVZ progenitors, contrasting the situation in the mouse cerebral cortex [20] , [21] , [34] , [35] . This difference is also reflected by the proportion of BPs expressing Tis21-GFP, an indicator of terminal neurogenic divisions [34] . While the vast majority of BPs in the cerebral cortex is Tis21-GFP+ [34] , [36] , it is rather a minority in the LGE ( Supplementary Fig. S3b ,c), further supporting the concept that only a minority undergoes terminal neurogenic divisions at mid-neurogenesis. An intriguing concept emerging from the possibility of proliferative divisions at all progenitor levels in the LGE is that the number of progeny may be adjusted at each of these stages in the lineage, that is, apically by regulating SNP–SNP divisions, subapically by regulating SAP–SAP divisions and at basal positions by regulation of BP–BP divisions. This may be a mechanism adapting neuronal output by varying signals from several sources at different developmental stages. RGs are only a subset of SAPs in the murine LGE, but they are special as only they generate bRGs, a key cell type required for gyrification, providing additional sources of neurons and RG guides to expand the cortical plate surface disproportional to the apical, ventricular surface [3] , [4] , [11] . Interestingly, this subset of bipolar RGs is particularly expanded in the cerebral cortex of species with a high GI and in the murine cerebral cortex upon Trnp1 knockdown. The latter results in more than 3 × increase in bRGs, the formation of an additional progenitor layer basal to the SVZ, reminiscent of the OSVZ, and even gyrus formation in the murine cerebral cortex [11] . Therefore these data support the concept that the bipolar RG subset serves in expanding SVZ progeny by generating bRGs in the gyrification process. Taken together, this novel progenitor cell has an important role in ontogeny and phylogeny. Animals C57BL/6J and Glast CreERT2 (ref. 37 ) crossed to Confetti reporter mice [26] were kept on a 12-h light–dark cycle. The day of the vaginal plug was considered as embryonic day (E) 0. Tamoxifen (5 μg g −1 bodyweight) was injected intraperitoneally. Animal experiments were performed according to the institutional and legal guidelines and were approved by the government of Upper Bavaria, the RIKEN Center for Developmental Biology, the Japanese government and by the local ethical review process ( http://www.nimr.mrc.ac.uk/animals-in-research/ethical-review-process/ ). IUE and plasmids IUEs were carried out on anaesthetized time-pregnant mice with the uterine horn constantly rinsed with Ringer solution (Braun) as described previously [36] . For short-term imaging, the plasmids pCIG2 (cytoplasmic GFP; gift from Dr C. Schuurmans) and pCAGGs-GAP43-GFP (ref. 38 ) were injected at a final concentration of 1 μg μl −1 each, together with Fast Green (2.5 μg μl −1 ; Sigma) into the lateral ventricles of the embryos, and electroporated with 5 pulses applied at ∼ 40 mV for 50 ms each at intervals of 100 ms by an ElectroSquireportator T830 (Harvard Apparatus). For long-term imaging, the plasmids pCAG-Floxp-EGFP-N1 and pCAG-Floxp-mKO2-F (both 0.5–0.8 μg μl −1 ) together with a low concentration of pCAGCre (0.05–0.3 ng μl −1 ) were electroporated with the same settings as above. The low concentration of Cre plasmid allowed sparse labelling of progenitor cells due to a recombination of a floxed stop cassette by the Cre recombinase in single cells, as also described in Shitamukai et al. [10] For labelling of cellular processes the plasmid pCAG-Floxp-EGFP-farnesylated (0.5–0.8 μg μl −1 ) was co-electroporated together with a low concentration of pCAGCre (8 ng μl −1 ). Slice culture imaging Slices of the embryonic telencephalon were cut at a thickness of 300 μm on a vibratome (Leica VT1200S or DSK) in ice-cold DMEM (Sigma) gased with oxygen (95%), immersed in a collagen-based matrix (Nitta Gelatin), covered with neurobasal medium with supplements and imaged in a gas (5% carbondioxide) floated wet chamber for short-term imaging ( Fig. 1 ; as also described in Asami et al. [36] ). For longer-term imaging ( Fig. 2 ; as also described in Shitamukai et al. [10] ) slices were embedded in the collagen matrix on a filter membrane (Millipore) and the medium consisted of DMEM-F12 (Sigma), 5% fetal calf serum, 5% horse serum, N2 supplement (1:100; Invitrogen), B27 supplement (1:50; Invitrogen), GlutaMax (1:100; Invitrogen), PenStrep (100 U ml −1 ). Imaging was performed on a confocal laser scanning microscope (FV1000, Olympus) using a 40 × long working distance objective (LUMPlanFl NA0.8, Olympus) and immersion oil for water dipping lenses (Immersol W; Zeiss). During imaging, slices were incubated in a stage-top incubator (Tokai Hit) at 37 °C in a 40% oxygen/5% carbondioxide atmosphere. The time interval between each time point was 20 min. In order to avoid the imaging of cellular artefacts, the first 20 μm of each slice were not recorded. In addition, brightfield images were taken at the same time to monitor the integrity of the slice. Immunohistochemistry Whole heads (E12) or mouse embryonic brains from the respective strains (E14–E16) were fixed in paraformaldehyde (PFA; 4% in PBS) for 1 (E12), 2 (E14) or 4 (E16) h. Brains were then either cryoprotected in 30% sucrose in PBS overnight and embedded in Tissue-Tek (Sakura) for sectioning at the cryostat (20–30-μm-thick), or embedded in 3% agarose (Biozym) in PBS for sectioning at the vibratome (70–100-μm-thick). Immunostaining on cryosections was performed by incubating the primary antibody overnight at 4 °C (in TBS with 0.5% Triton-X and 10% normal goat serum), while the vibratome sections were incubated longer (for 2 days, due to the larger thickness of the sections), with the primary antibodies used at the following concentrations: anti-Ascl1 (Developmental Hybridoma Bank, IgG1, 1:200), anti-βIII-tubulin (Sigma, mouse IgG2b, 1:200), anti-GFP (Sigma, chicken, 1:1,000), anti-Glast (Chemicon, Guinea pig, 1:400), anti-Islet1 (Hybridoma Bank, IgG2, 1:50), anti-Pax6 (Chemicon, rabbit, 1:400), anti-pericentrin (Covance, rabbit, 1:1,000), anti-phosphorylated histone H3 (Biomol, rabbit, 1:400), anti-Dlx2 (Millipore, rabbit, 1:200), anti-p-vimentin (MBL, mouse IgG2b, 1:500) RC2 (mouse, IgM, 1:500, kind gift of P. Leprince) and the Sox2 antibody (Millipore, rabbit, 1:500). After washing three times with PBS, sections were incubated with the respective fluorochrome-labelled secondary antibodies overnight, washed again, incubated in DAPI (1/1000; Sigma) and embedded after further washes in Aqua Polymount (Polyscience). Images were taken and analysed using a FV1000 confocal laser scanning microscope (FV1000; Olympus). Pigmented ferrets ( Mustela putorius furo ) were obtained from Marshall Farms (North Rose, NY) and kept on a 12:12-h light:dark cycle at the Animal Facilities of the Universidad Miguel Hernández, where animals were treated according to the Spanish and EU regulations, and experimental protocols were approved by the Universidad Miguel Hernández IACUC. Viral injections were performed 24 h after the ferrets were born, on individuals of both sexes. Live sheep embryos of both sexes were obtained from the slaughter house MURGACA (Cartagena, Spain) with permission, and under the supervision of the veterinary in chief. The age of the collected embryos was determined a posteriori based on the crown-rump length as described [39] . Measurements on sheep embryos were carried out before perfusion. Fixed embryonic brains of common marmoset ( Callithrix jacchus; no sex preference) were obtained from the Wisconsin National Primate Center in Madison, WI, USA. The stage of pregnancy was determined on the basis of breeding time and embryo size. Single and double immunostains were performed on 50-μm-thick free-floating sections. Sections were blocked and incubated in the following primary antibodies overnight at 4 o C: anti-phosphohistone 3 (1:1,000, Upstate), anti-phosphovimentin (1:1,000, Abcam), chicken anti-GFP (1:1,000, Aves) and anti-Ascl1 (1:500, Abcam). Sections were then incubated with appropriate fluorescently conjugated secondary antibodies (Chemicon and Jackson) and counterstained with DAPI (SIGMA). Confocal images were acquired using a confocal spectral microscope Leica SP2 AOBS, taken as 0.8-μm ( × 40) single optical sections, which were then compressed using their maximum projection. Conventional fluorescence microscopy images were obtained using a Leica CTR5000 microscope. Cortical layers were determined as described in Reillo et al. [9] and Kelava et al. [28] Shortly, the VZ was defined as the pseudostratified epithelial layer with constant thickness. The ISVZ lies basally to the VZ, also has a high cell density but no columnar organization. The OSVZ is defined as the columnar cell-sparse layer basal to the ISVZ-containing proliferating cells. The intermediate zone (IZ) is a layer of very low density with virtually no mitotic cells, including the subplate (SP). The cortical plate (CP) was defined as the high-dense layer located between IZ and mantle zone (MZ), including the already formed layers 5 and 6. PH3+ and Ph-Vim+ cells were counted from rectangular sectors of the cortex spanning its entire thickness, using Neurolucida and Neurolucida Explorer software (Microbrightfield). G fp -encoding Retrovirus (Rv: gfp ) and Adenovirus (Adeno: gfp ) stocks were injected in the outer SVZ and cortical plate, respectively, of the postnatal ferret kits, as described previously [9] . Shortly, the ferret kits were deeply anaesthetized with isoflurane 1.5%. Two microlitres of Rv: gfp was injected into the OSVZ. The Adeno: gfp was injected into the CP at the age of P4 in several locations to amplify the labelling. All these injection sites were defined by stereotaxic coordinates and the operations were approved by the Universidad Miguel Hernández IACUC All kits were overdosed with pentobarbital and perfused with 4% PFA, and brains were postfixed overnight. Free-floating sections (50 μm thickness) were obtained by cryotome sectioning. How to cite this article: Pilz, G.-A. et al. Amplification of progenitors in the mammalian telencephalon includes a new radial glial cell type. Nat. Commun. 4:2125 doi: 10.1038/ncomms3125 (2013).